Rational strategy for shaped nanomaterial synthesis in reverse micelle reactors The shape-controlled synthesis of nanoparticles was established in single-phase solutions by controlling growth directions of crystalline facets on seed nanocrystals kinetically; however, it was difficult to rationally predict and design nanoparticle shapes. Here we introduce a methodology to fabricate nanoparticles in smaller sizes by evolving shapes thermodynamically. This strategy enables a more rational approach to fabricate shaped nanoparticles by etching specific positions of atoms on facets of seed nanocrystals in reverse micelle reactors where the surface energy gradient induces desorption of atoms on specific locations on the seed surfaces. From seeds of 12-nm palladium nanocubes, the shape is evolved to concave nanocubes and finally hollow nanocages in the size ~10 nm by etching the centre of {200} facets. The high surface area-to-volume ratio and the exposure of a large number of palladium atoms on ledge and kink sites of hollow nanocages are advantageous to enhance catalytic activity and recyclability. Previously, the evolution of the size of spherical inorganic nanoparticles (NPs) via atomic adsorption/desorption processes has been rationally established in one-phase solutions [1] , [2] , [3] , [4] , [5] , [6] . The size-dependent solubility of NPs in the solution is illustrated by the Gibbs–Thomson equation [7] : where S r and S ∞ are solubility of the NP and its bulk counterpart, σ is the specific surface energy, V m is the molar volume of NPs, r is the particle radius, R is the gas constant and T is the absolute temperature. In the condition of particle growth under a given precursor concentration ( S b ), an equilibrium particle radius ( r *) is derived from Equation 1 [7] : To correlate the size change of NPs and ion concentration in solution for predicting the shape evolution of NPs in a typical diffusion control growth reaction, d(Δ r )/d t is derived as: where Δ r is the s.d. of size distribution, K D is a constant and is the mean radius of NPs [7] . From these equations, three important factors to control atomic adsorption on seed nanocrystals can be derived: (1) ion precursor concentration in solution, (2) distribution of high/low surface energy of crystalline facets on seeds and (3) topological shape of seeds. To promote the particle growth in the narrow size distribution with atomic adsorption, it is important to maintain the condition where the precursor concentration is relatively high because /2 in Equation 3 needs to be larger than r * and r * monotonically decreases with increasing S b in Equation 2 (ref. 1 ). On the contrary, etching and desorption mode of atoms from the seed NPs becomes thermodynamically favourable when the precursor concentration is low (that is, < r *), which is the scope of this work. In addition, the surface energy is also important to determine adsorption/desorption of atoms from specific crystalline facets of seeds; when surface atoms on seed nanocrystals are exposed to solution under the minimal influence of capping agents (that is, low coverage and disorder of capping structures), desorption of atoms on high-energy crystalline facets is promoted while re-adsorption could become more dominant on low-energy crystalline facets, dependent upon the reactivity of desorbed species. Owing to this feature, the surface energy landscape created by the distribution of facets displaying distinct surface energy can direct the shape evolution of seeds. Furthermore, the topological shape of seed nanocrystals can also affect the thermodynamic adsorption/desorption of atoms on surfaces. For example, Equation 1 shows that the solubility of atoms from the crystalline facet is dependent on the geometric curvature of the NPs ( r in Equation 1). It means that atoms on concave surfaces have distinct desorption property as compared with flat and convex surfaces [8] . Thus, the application of shaped nanocrystals as seeds gives one a new toolbox for designing NPs in complex structures by controlling atomic adsorption/desorption in more precise patterns. In addition, fabricating NPs in complex shapes by optimizing three factors for the shape evolution from seed nanocrystals leads to rationale pathways for designing novel NPs. While polyhedron-shaped NPs are dominant for the use as seeds via reduction of ionic precursors [9] , spherical seeds delocalize the surface energy landscape and thus the shape evolution tends to be simply dependent on the distribution of crystalline faces. Since the number of displayed crystalline faces is limited on the spherical nanocrystals, it is desirable to use the faceted seed nanocrystals for more delocalized surface energy distribution if the shape needs to be rationally evolved into more complex structures through atomic adsorption/desorption [10] . Fortunately, seeds are now available in a variety of non-spherical shapes with high monodispersity because of the recent progress in shape-controlled NP synthesis [11] , [12] , [13] , [14] , [15] , [16] , [17] . As explained above, the advantage for the use of non-spherical seed nanocrystals is to add predictable surface energy gradient based on their shape. Previously, various shaped NPs were grown by adsorbing atoms on low-energy facet of the seed nanocrystals in high precursor concentration [18] , [19] , [20] , [21] , [22] , [23] , [24] , [25] , [26] , [27] , [28] , [29] , [30] . A one-pot solvothermal method was also applied to synthesize concaved platinum (Pt) nanoframes by mediating the concentration of capping agent [31] . Through the atomic adsorption approach, concaved palladium (Pd) nanocubes were also grown by adsorbing Pd atoms kinetically on {111} facets while high-energy {200} facets were capped ( Fig. 1a ) [32] . These approaches are suitable to grow large sized NPs; however, it is difficult to produce concave and hollow NPs in the size smaller than 15 nm since the size and quality of seeds limit the final dimension via the atomic adsorption mode [31] , [32] . To fabricate smaller shaped NPs, chemical etchants were used to etch atoms on high-energy facets; however the use of etchants makes the etching reaction chemistry complicated, sensitively dependent on the type of etchants and their concentration, and the interfacial dynamics of capping agents on selected crystalline facets also adds another complexity [33] , [34] , [35] , [36] , [37] , [38] , [39] . Previously, the shape of gold (Au) NPs was transformed from nanorods to nanospheres by desorbing capping agents by heating because atoms on the high-energy surface migrate to lower surface energy facet [40] . The aspect ratio of cadmium selenide (CdSe) nanorods was also changed by transferring surface atoms to lower surface energy facets through the interparticle ripening route [41] . These strategies for nanosphere and nanorod growth inspired us to design more complex-shaped NPs using the rational synthesis pathway by balancing the surface energy landscape and the topological shape of seed nanocrystals: if the seed nanocrystals display well-defined surface energy distribution among crystalline facets, the resulting shape of nanocrystals after atomic desorption is predictable. 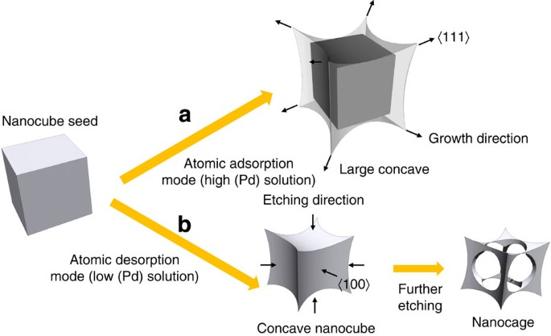Figure 1: Shape evolution mechanisms. Evolution processes of nanocubes into the concaved shape via (a) a traditional growth approach with atomic adsorption on selected facets (b) an approach in this work with atomic desorption on selected facets. Figure 1: Shape evolution mechanisms. Evolution processes of nanocubes into the concaved shape via ( a ) a traditional growth approach with atomic adsorption on selected facets ( b ) an approach in this work with atomic desorption on selected facets. Full size image In this work, the shape of 12-nm Pd seed nanocubes is evolved to concave nanocubes and finally hollow nanocages in the size ~10 nm by etching specific positions of atoms on facets of seed nanocrystals based on the surface energy distribution in reverse micelle reactors ( Fig. 1b ). The high surface area-to-volume ratio and the exposure of a large number of Pd atoms on ledge and kink sites of hollow nanocages enhance catalytic activity and recyclability in Suzuki coupling reactions. Structural evolution from nanocube to nanocage The etching strategy is summarized in Fig. 2a . In step (i), the seeds of Pd nanocubes are dispersed in aqueous compartment of reverse micelle. The Pd nanocube seeds are hydrophilic as their {200} facets are protected by a well-defined bilayer of cetyltrimethylammonium bromide (CTAB; Fig. 2ai ) [24] , [26] , [42] , [43] , [44] . Next, in step (ii), heating slowly evaporates the water phase. In step (iii), the hydrophilic compartment becomes smaller and eventually transformed into one single layer of CTAB whose polar headgroups directly contact the well-defined bilayer of CTAB on Pd NPs, and then diffusion of the organic solvent destabilizes this capping structure. In step (iv), reduction in coverage and disorder in the packing structure of capping agents occur more dominantly at the centre of {200} facets. As a result, desorption of Pd atoms from the surface of seeds is triggered because of the surface energy gradient. In addition, the formation of stable Pd complexes between desorbed Pd atoms and CTAB in solution further promotes the release of Pd atoms and discourages the re-adsorption of Pd atoms on the seeds. This strategy enables the localized etching of Pd atoms on the nanocube seeds, and it creates concaved nanocubes and then the shape is further evolved into nanocages as shown in Fig. 2b . 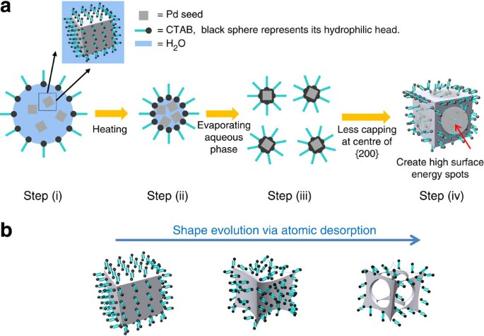Figure 2: Shape evolution of seed nanocrystals in reverse micelle reactors. (a) Scheme for the shape evolution of Pd NPs. Step (i): seeds of Pd nanocubes are dispersed in aqueous compartment of reverse micelle. Step (ii): slow evaporation of water phase. Step (iii): diminishing water phase induces partial removal of capping agents in octanol. Step (iv): gradients of surface energy on shaped seed nanocrystals with localized capping lead to atomic desorption at high surface energy area on the seed NPs. (b) The etching of seed nanocubes takes place at the centre of {200} facets because of the surface energy landscape in the step (iv). The evolution of shapes follows from concave nanocubes to nanocages with etching time. Figure 2: Shape evolution of seed nanocrystals in reverse micelle reactors. ( a ) Scheme for the shape evolution of Pd NPs. Step (i): seeds of Pd nanocubes are dispersed in aqueous compartment of reverse micelle. Step (ii): slow evaporation of water phase. Step (iii): diminishing water phase induces partial removal of capping agents in octanol. Step (iv): gradients of surface energy on shaped seed nanocrystals with localized capping lead to atomic desorption at high surface energy area on the seed NPs. ( b ) The etching of seed nanocubes takes place at the centre of {200} facets because of the surface energy landscape in the step (iv). The evolution of shapes follows from concave nanocubes to nanocages with etching time. Full size image Pd nanocubes for seeds The Pd nanocubes were prepared in an aqueous solution at 95 °C. After sodium tetrachloropalladate(II) (Na 2 PdCl 4 ), sodium hydroxide (NaOH) and CTAB were dissolved in water and stirred vigorously at 95 °C and freshly prepared ascorbic acid solution was immediately injected into the reaction system. The reaction was kept at 95 °C for 30 min. The product was collected using centrifugation and was washed with water. Transmission electron microscopy (TEM) image shows that as-prepared Pd nanocubes have an average size and the size distribution of 12 nm and <10%, respectively ( Supplementary Figs 1a and 2 ). High-resolution TEM (HRTEM) image reveals the single crystal characteristics of the nanocubes with the lattice fringe spacing at 2.0 Å, corresponding to the {200} planes of face centred cubic (fcc) Pd ( Supplementary Fig. 1b,c ). The inset in Supplementary Fig. 1b is the indexed fast Fourier transform (FFT) pattern of Supplementary Fig. 1b , consistent with the single crystalline pattern of the Pd nanocubes. Generation of Pd nanocages by etching Pd nanocube seeds The etching treatment was conducted in a reverse micelle system made of CTAB/octanol/H 2 O. In 20 min after residual octanol and excess surfactants were removed by washing with ethanol and water, the edges of Pd NPs were excavated on six faces, while the overall size remained the same as Pd seeds ( Fig. 3a ). HRTEM image of the Pd concave nanocube in Fig. 3b reveals darker contrasts at the corners, indicating that the sample is thicker at the corners and is thinner in between after the etching treatment. The single crystal characteristics observed along the [100] axis is demonstrated by the corresponding FFT pattern in the inset of Fig. 3b . 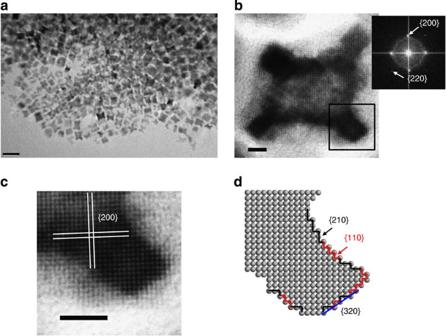Figure 3: Structural analysis of Pd nanoconcave crystals. (a) TEM and (b) HRTEM images of the Pd concave nanocubes fabricated after 20 min of etching (inset: the FFT pattern). Scale bar=20 nm inaand 2 nm inb, respectively. (c) Magnified image of the square region highlighted inb. Scale bar=2 nm. (d) Atomic modelling corresponding to the region inc, where the {110} and {210} subfacets are marked with red and black, respectively. A high-index {320} plane that is composed of alternating {110} and {210} is labelled with blue. Figure 3c shows higher magnification of the corner region highlighted of a squared area in Fig. 3b . A large number of surface atoms are situated at ledge, ledge–kink and kink sites after etching, and it generates complex lattice fringe patterns on the surface. Figure 3d shows the two-dimensional (2D) lattice modelling corresponding to Fig. 3c , where a high-index {320} plane (marked in blue) composed of alternating subfacets of {110} (marked in red) and {210} (marked in black) is tentatively labelled. This result indicates that CTAB cannot completely protect these nanocrystals, and desorption of Pd atoms from the seed is predominant while the rate of re-adsorption on lower-energy surfaces is negligible at this early stage of shape evolution. This sparse growth may be attributed to the low concentration of and the low reactivity of Pd species in the hydrophobic solution. Figure 3: Structural analysis of Pd nanoconcave crystals. ( a ) TEM and ( b ) HRTEM images of the Pd concave nanocubes fabricated after 20 min of etching (inset: the FFT pattern). Scale bar=20 nm in a and 2 nm in b , respectively. ( c ) Magnified image of the square region highlighted in b . Scale bar=2 nm. ( d ) Atomic modelling corresponding to the region in c , where the {110} and {210} subfacets are marked with red and black, respectively. A high-index {320} plane that is composed of alternating {110} and {210} is labelled with blue. Full size image After 1 h of further etching treatment, the concaved nanocubes were transformed into hollow nanocages ( Fig. 4a ). 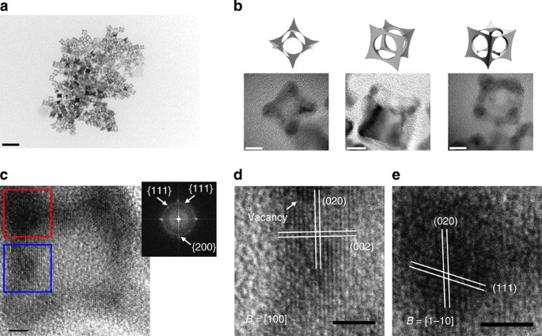Figure 4: Structural analysis of Pd nanocages. (a) A low-magnification TEM image to show the overall morphology of the products. Pd nanocages were generated after 1 h of etching. Scale bar=50 nm. (b) High-magnification TEM images of individual nanocages in various angles. Scale bars=5 nm. (c) A HRTEM image of the nanocage (inset: the FFT pattern). (d) A magnified image of the edge region highlighted with a blue square inc. (e) A magnified image of the corner region highlighted with a red square inc.Bdenotes the beam direction indande. Scale bars=2 nm inc–e. Figure 4b shows TEM images of individual nanocages at different angles. The average edge length of nanocage is 10 nm, 2 nm shorter than the one for the seed ( Supplementary Fig. 2 ). It suggests that atoms on the corners of seeds started to dissolve into the solution at this aging time. The hollow structure of Pd nanocage was also confirmed from a series of TEM images obtained through tilting the sample stage at a variety of angles ( Supplementary Fig. 3 ). The nearly pure composition of Pd of the nanocage was confirmed using the energy-dispersive X-ray spectrum ( Supplementary Fig. 4 ). While the nanocages are single crystalline in general ( Supplementary Fig. 5 ), some NPs show polycrystalline characteristics. As shown in the HRTEM image of Fig. 4c and its corresponding inverse FFT images ( Supplementary Fig. 6 ), the edges of the nanocages are imaged along [100], where the (020) and (002) planes of fcc Pd are indexed. Meanwhile, the left upper corner area of the nanocages is imaged along [1–10], and lattice fringes corresponding to (020) and (111) planes of fcc Pd are resolved. A vacancy separating these two crystalline zones is marked with an arrow in Fig. 4d . The polycrystalline characteristics are also confirmed by the FFT pattern in the inset of Fig. 4c , where a superposition of [100] and [1–10] zones are indexed. The observation of shape transformation from nanocubes to concave nanocubes and finally hollow nanocages indicates that the shape evolution occurs thermodynamically so that the etching patterns are consistent with surface energy landscape created by the reorganization of capping agents in the diminishing reverse micelle compartment. The observation of atomic re-adsorption on the lowest-energy {111} facets [45] with complicated lattice fringes with atoms on ledge, ledge–kink and kink sites ( Fig. 4c ) becomes more noticeable after 1 h of the shape evolution, probably because of the increased concentration of Pd in solution inducing their re-adsorption on these sites. Figure 4: Structural analysis of Pd nanocages. ( a ) A low-magnification TEM image to show the overall morphology of the products. Pd nanocages were generated after 1 h of etching. Scale bar=50 nm. ( b ) High-magnification TEM images of individual nanocages in various angles. Scale bars=5 nm. ( c ) A HRTEM image of the nanocage (inset: the FFT pattern). ( d ) A magnified image of the edge region highlighted with a blue square in c . ( e ) A magnified image of the corner region highlighted with a red square in c . B denotes the beam direction in d and e . Scale bars=2 nm in c – e . Full size image As illustrated in Fig. 2a , the shape evolution of seed nanocubes is driven by the structure change of capping layers on seed nanocrystals after water compartment is evaporated in the reverse micelle system. To probe the packing condition of CTAB capped on shaped NPs, Fourier transform infrared spectroscopy is applied to Pd nanocubes before and after etching, where peak positions and widths of C-CH 2 asymmetric and symmetric stretching vibrations of the methylene chain of CTAB can be used to assess the nature of surfactant packing on solid surfaces [40] , [46] . In Supplementary Fig. 7 , as compared with the crystalline CTAB, both stretching vibrations shift to the higher frequency for CTAB-capped Pd nanocubes (from 2,917 to 2,920 cm −1 for the asymmetric band and from 2,849 to 2,851 cm −1 for the symmetric band). The lower vibrational frequency and the narrower bandwidth for the crystalline surfactant correspond to more ordered structures of the methylene chains of CTAB [40] , [46] . Since the stretching bands for CTAB on Pd nanocubes are blue-shifted relative to crystalline CTAB and their frequencies are comparable to the ones on gold nanorods (2,921 and 2,851 cm −1 , respectively), CTAB forms a well-defined bilayer capped on Pd nanocubes with less degree of packing order than the crystalline state [38] . As both symmetric and asymmetric bands for CTAB on Pd nanocages are further shifted to 2,922 cm −1 and 2,853 cm −1 , respectively ( Supplementary Fig. 7 ), it indicates that CTAB covers the surface of Pd nanocages with less packing order and surface coverage as compared with Pd nanocubes, yielding a large number of less-protected surface atoms exposed at ledge, ledge–kink and kink sites [40] , [46] , consistent with nanoscopic structures in Fig. 4c . Effect of solvents on atomic desorption In addition to the effect of the surface energy distribution, desorption of Pd atoms from the seed nanocrystals could be promoted by the formation of stable Pd complexes between desorbed Pd atoms and solute molecules. To confirm this hypothesis, we carried out UV–vis absorption measurements of solution during the shape evolution process. Under the experimental condition, Pd atoms dissolved from {200} facets in octanol can readily oxidized into CTA + [PdX 4 ] 2− complex species (X=Cl or Br) [24] , [47] , and a minute amount of the oxidized forms of ascorbic acid residue (for example, semidehydroascorbic acid and dehydroascorbic acid) in the Pd seed solution may serve as oxidants. After 1 h of etching and separation of Pd NPs with centrifugation, the remaining supernatant was analysed. While octanol solution containing only CTAB (20 mg ml −1 ) shows no absorption peaks, the spectrum of supernatant shows two peaks at 250 and 340 nm, respectively ( Supplementary Fig. 8a ). Both peaks are corresponded to the ones for CTA + [PdX 4 2− ] complex ions [47] . A series of UV–vis spectra of CTA + [PdX 4 2− ] with the concentration ranging from 0 to 180 μM in octanol also showed the similar absorption profile ( Supplementary Fig. 8b ), and they follow the Beer–Lambert law as shown in Supplementary Fig. 8c . This result suggests that the desorbed individual Pd atoms are highly reactive in solution and they can readily be oxidized and can form the stable complex during the etching treatment. Since the relatively high stability of complexes between Pd atoms and solute molecules promotes the desorption of Pd atoms from Pd nanocubes, types of solvents should also influence the etching process. As shown in Supplementary Fig. 9a , when the seeds were aged in ethylene glycol, a polar solvent, instead of octanol, NPs were grown in larger sizes while maintaining their cubic shape, indicating that the bilayer capping of CTAB on {200} facets was intact. As no obvious etching was observed on the seed nanocrystals, the reaction rates of dissolving of small NPs and the growth of large NPs are equally high and large NPs grow at the expense of smaller seeds as seen in Ostwald ripening. The faster crystal growth in EG is attributed to the higher reactivity of CTA + [PdX 4 ] 2− in the polar solvent [48] , [49] . When the reaction was conducted in a 1:1 EG/octanol solution, normal Ostwald ripening was still observed; however, NPs no longer maintained their cubic shape ( Supplementary Fig. 9b ). Adding octanol to EG solution increased the hydrophobicity of the solution, and it seems to destabilize the bilayer structure of CTAB on {200} facets of Pd nanocubes so that the shape of NPs became irregular after aging at elevated temperature. Catalytic performance and mechanism As the hollow Pd nanocages have the large surface area-to-volume ratio and they also exhibit the high density of catalytically active atoms on the ledge, ledge–kink and kink sites, these characteristics prompted us to investigate their potential catalytic performance. To this end, the catalytic activities of 10-nm Pd nanocages and 12-nm Pd nanocubes were compared in Suzuki coupling reactions. First, the coupling between phenylboronic acid (PhB(OH) 2 ) and iodobenzene was investigated in 80% ethanol aqueous solution at room temperature. As shown in Fig. 5a , Pd nanocages show superior catalytic property that a nearly complete formation (>90%) of C–C bond is achieved within 30 min, whereas 12-nm Pd nanocubes can only promote a conversion of ~40% under the same condition and it required 75 min to reach a steady conversion of ~80%. In Fig. 5b , Pd nanocages also demonstrate excellent recycling performance while small loss of catalytic property is observed for Pd nanocubes after circles of the reuse. The cumulative turnover number (mol of product/mol Pd) over six runs for Pd nanocages (10 μg, 0.03 mol%) is 1.9 × 10 4 , which is 1.3 times higher than the one for the Pd nanocubes. To compare them in more difficult catalytic environment, iodobenzene is replaced by iodotoluene, an electron-neutral aryl iodide, which is less reactive in the coupling reaction [50] , [51] . As shown in Fig. 5c , the reaction catalysed by Pd nanocages was nearly completed (>90%) after 90 min, while Pd nanocubes could convert only <30% of reactants at 50 °C. In this harder coupling reaction between PhB(OH) 2 and iodotoluene, the turnover number for Pd nanocages (10 μg, 0.03 mol%) remains 1.9 × 10 4 over six runs; however, it is 4.5 times higher than the one for Pd nanocubes, and the superior recyclability for Pd nanocages over Pd nanocubes is also demonstrated ( Fig. 5d ). It should be noted that no homocoupled product was observed during the coupling between PhB(OH) 2 and iodotoluene, as supported by nuclear magnetic resonance (NMR) spectra ( Supplementary Fig. 10 ). 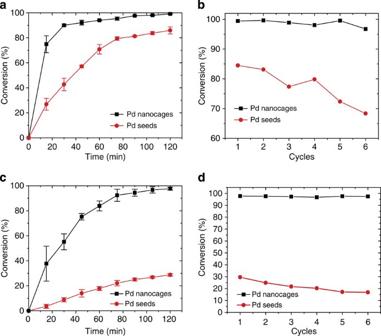Figure 5: Catalytic performance of the Pd NPs in Suzuki coupling reaction. For the coupling reaction between phenylboronic acid and iodobenzene at room temperature: (a) catalytic conversion % by 12-nm Pd nanocubes and 10-nm Pd nanocages, respectively. (b) Comparison of recyclability between the Pd nanocube catalyst and the Pd nanocage catalyst. For the coupling reaction between phenylboronic acid and iodotoluene at 50 °C: (c) catalytic conversion % by 12-nm Pd nanocubes and 10-nm Pd nanocages, respectively. (d) Comparison of recyclability between the Pd nanocube catalyst and the Pd nanocage catalyst. The reaction time is 120 min. Ina,c, error bars represent the s.d. (n=3). Figure 5: Catalytic performance of the Pd NPs in Suzuki coupling reaction. For the coupling reaction between phenylboronic acid and iodobenzene at room temperature: ( a ) catalytic conversion % by 12-nm Pd nanocubes and 10-nm Pd nanocages, respectively. ( b ) Comparison of recyclability between the Pd nanocube catalyst and the Pd nanocage catalyst. For the coupling reaction between phenylboronic acid and iodotoluene at 50 °C: ( c ) catalytic conversion % by 12-nm Pd nanocubes and 10-nm Pd nanocages, respectively. ( d ) Comparison of recyclability between the Pd nanocube catalyst and the Pd nanocage catalyst. The reaction time is 120 min. In a , c , error bars represent the s.d. ( n =3). Full size image It is unlikely that leaching Pd atoms from Pd nanocages catalyse the Suzuki coupling reaction between aryl iodide and PhB(OH) 2 in Fig. 5 because if Pd atoms are released from Pd nanocages as homogeneous catalysts, deformation of the shape of nanocages along with declined catalytic turnovers should be observed in the recycling process even though some of these Pd atoms are readsorbed on the nanocage. To firmly confirm that no leaching Pd species are involved in the Suzuki coupling reaction, the three-phase test was examined under the standard condition (0.6 mmol PhB(OH) 2 , 0.3 mmol iodobenzene or iodotoluene, 1 mmol K 2 CO 3 , 10 μg Pd nanocages (0.03 mol%) and 5 ml 80% ethanol aqueous solution) in the presence of NovaSyn TGR resin-supported aryl iodide ( 2 in Supplementary Fig. 11 ) [52] , [53] . While the quantitative recovery of biphenyl products was still achieved in the solution phase, no biphenylamide ( 6 in Supplementary Fig. 11 ) was detected after cleavage of the resin with trifluoroacetic acid (TFA) by gas chromatography–mass spectrometry (GC–MS) and NMR ( Supplementary Figs 12 and 13 ). Thus, these results indicate that no free Pd atoms or Pd-organic complexes are involved in the Suzuki coupling reactions in the aqueous solution at relatively low reaction temperature, and the catalytic reactions only take place on the surface of Pd nanocages [54] . The heterogeneous catalytic nature of Pd nanocages indirectly supports the hypothesis above that the superior catalysis is related to the large number of active Pd atoms exposed on the surface. The dominant desorption of Pd atoms from the centre of {200} facets leads to fabrication of hollow NPs with concaved framework, in the size ~10 nm, less than the one for the seeds. While the overall sizes of individual NPs were decreased relative to seeds in this anisotropic etching treatment, the size distribution was not notably changed because of the survival of low-energy facets on seeds. To turn on the atomic desorption mode for etching, the well-defined packing structures of capping agents were disordered and their coverage on NPs was reduced via interference with organic solvent after the aqueous compartment of reverse micelle was evaporated ( Fig. 2a(ii) and (iii) ). Consequently, the surface energy gradient was generated, which could trigger the etching on specific locations on the seed surfaces ( Fig. 2a(iv) ). To examine whether this approach can be applicable to generate other shaped metal NPs, Au nanocages were synthesized by etching Au nanocube seeds with the same method used for the synthesis of Pd nanocages. The three-dimensional (3D) characteristics of hollowness of Au nanocages were verified with their TEM images at different tilt angles ( Supplementary Fig. 14 ). Thus, this experiment suggests that the atomic desorption-based etching approach can be widely applicable to fabricate a variety of shaped NPs with the simple etching mechanism. In conclusion, the seed-etching nanofabrication approach for the shape-controlled NPs was designed and demonstrated. The shape evolution from the seed nanocubes to concave nanocubes and finally hollow nanocages were observed by controlling atomic desorption from specific areas of the seed surfaces. The shape evolution occurred thermodynamically, and the etching patterns were consistent with surface energy landscape created by the structure change of capping layers in reverse micelle reactors. The stability of ion complexes between desorbed Pd ions and solute molecules was also important to promote the atomic desorption mode on the seed nanocubes. The seed-etching process sheds light on the rational design of shape-controlled synthesis of NPs. In addition to the demonstration of Pd and Au nanocage fabrications in reverse micelle reactors in this work, very recently the shape evolution was applied for fabricating platinum–nickel (Pt–Ni) bimetallic nanoframes by preferentially eroding Ni atoms distributed towards the interior of polyhedral faces of seed nanocrystals via oxidation [55] . Therefore, the shaped NP fabrication via the atomic etching strategy on selected positions of seeds is versatile and it is expected to have broad impacts on a variety of nanotechnological applications. This fabrication strategy will be beneficial for a variety of areas such as catalysis [56] , plasmonics [17] , [57] , electronics [58] , [59] and biomedicine [60] , [61] , [62] where rational shape-controlled synthesis of NPs in size <20 nm has significant impact on their performances [17] , [45] , [58] , [63] . For catalysis, such small complex-shaped NPs are expected to have high catalytic activity because the complex hollow structures of Pd nanocages exhibit a large number of atoms on ledge, ledge–kink and kink sites with high surface areas [64] , [65] , [66] , [67] , [68] . Chemicals Sodium tetrachloropalladate(II) (Na 2 PdCl 4 , 99.995%), gold(III) chloride hydrate (HAuCl 4 , ≥9% Au basis), sodium hydroxide (NaOH, ≥8%), sodium borohydride (NaBH 4 , ≥99%), CTAB (≥99%), ascorbic acid (≥99.0%), 1-hydroxybenzotriazole hydrate (HOBt, 99%), N,N ′-diisopropylcarbodiimide (DIC, 99%), acetic anhydride (Ac 2 O, 99.5%), ethanol (≥99.5%), methanol (MeOH, ≥99.5%), 1-octanol (≥99%), dichloromethane (CH 2 Cl 2 , ≥99.9%), ethyl acetate (EtOAc, 99.8%), tetrahydrofuran (THF, ≥99.9%), EG (≥99%), N,N -dimethylformamide (DMF, ≥99%), pyridine (≥99.9%), iodobenzene (98%), 4-iodotoluene (≥99%), 4-iodobenzoic acid (98%), biphenyl-4-carboxamide (96%), phenylboronic acid (PhB(OH) 2 , >98%), deuterated chloroform (CDCl 3 , 99.8%), deuterated dimethyl sulfoxide (DMSO-d6, 99.9%), TFA (≥99.0%), potassium carbonate (K 2 CO 3 , ≥99.0%) and magnesium sulphate (MgSO 4 , ≥99.5%) were all purchased from Sigma-Aldrich, and were used as received without further purification except THF, which was distilled to remove butylated hydroxytoluene (BHT). NovaSyn TGR resin (0.25 mmol g −1 loading) was purchased from EMD Millipore. Sartorius ultrapure water (18.2 MΩ cm) was used in all preparations. Synthesis of Pd nanocubes The 12-nm Pd nanocube seeds were synthesized in the modified method on the basis of report by Niu et al. [14] , [43] Typically, 600 μl of 30 mM Na 2 PdCl 4 solution and 200 μl of 500 mM NaOH were added to 10 ml of 12.5 mM CTAB solution under stirring. After the solution was heated at 95 °C for 10 min, 200 μl of freshly prepared 500 mM ascorbic acid solution was added. The reaction was allowed to proceed for 30 min. Then, the product was separated using centrifugation and washed with water. The as-prepared Pd seeds were stored in water at 4 °C. Synthesis of Au nanocubes Au nanocubes were synthesized using the seed-mediated method according to Chen et al. [69] In a typical seed synthesis, a freshly prepared, ice-cold aqueous NaBH 4 solution (0.01 M, 0.3 ml) was added into an aqueous mixture solution composed of HAuCl 4 (0.01 M, 0.125 ml) and CTAB (0.1 M, 3.75 ml). The solution was mixed by rapid inversion for 2 min, and then kept at room temperature for 1 h before use. In a typical growth reaction, CTAB (0.1 M, 6.4 ml), HAuCl 4 (0.01 M, 0.8 ml) and ascorbic acid (0.1 M, 3.8 ml) were sequentially added into H 2 O (32 ml). Twenty microlitres of the CTAB-stabilized seed solution were diluted 10 times with water and then added into the growth solution. The resulting solution was mixed by gentle inversion for 10 s and then left undisturbed overnight. The product was separated using centrifugation and washed with water. The as-prepared Au nanocubes were stored in water at 4 °C and used as seeds for the etching experiment. NP etching The seed-etching treatment was conducted under argon (Ar) to avoid oxidation of Pd into PdO. In the typical experiment, an aqueous Pd seed solution (1 mg ml −1 , 200 μl) was added into octanol containing CTAB (20 mg ml −1 , 5 ml). A clear reverse micelle system made of CTAB/octanol/H 2 O was formed with stirring and ultrasonic treatment, where Pd seed NPs were dispersed in the water phase. Subsequently, the solution was heated to 105 °C to evaporate water in the reverse micelles with bubbling of Ar. It should be noted that no additional etchant was added into the reaction system. A set of products in a variety of shapes with different etching time was collected using centrifugation and washed with ethanol twice, and then water was added three times to remove residue oil and excess surfactants. The products were stored in water at 4 °C. The etching treatment for Au nanocubes follows the similar procedure as for Pd. Specifically, an aqueous Au nanocube solution (0.2 mg ml −1 , 200 μl) was added into octanol containing CTAB (20 mg ml −1 , 5 ml). The solution was heated to 105 °C to evaporate water in the reverse micelles with bubbling of Ar. After 1 h, the products were collected using centrifugation and washed with ethanol twice and then water three times to remove residue oil and excess surfactants. The products were stored in water at 4 °C. Catalytic evaluation in Suzuki coupling reactions Suzuki coupling reaction was performed according to procedures in previous reports [32] , [70] . For the catalytic synthesis of biphenyl compounds, PhB(OH) 2 (73 mg, 0.6 mmol) was added to ethanol (4 ml) with iodobenzene (34 μl, 0.3 mmol) or iodotoluene (65 mg, 0.3 mmol) in the presence of K 2 CO 3 (138 mg, 1 mmol) and aqueous solutions containing Pd NPs (1 ml, 10 μg ml −1 , 0.03 mol%). Reactions were carried out under vigorous stirring at room temperature for iodobenzene and 50 °C for iodotoluene, respectively. The biphenyl product and unreacted aryl iodides (if any) were extracted with CH 2 Cl 2 (3 × 5 ml), while the excess PhB(OH) 2 and Pd NPs remained in the aqueous layer [64] . The organic layer was then washed with saturated K 2 CO 3 solution three times, and it was dried over MgSO 4 powders. After filtration, CH 2 Cl 2 was removed through rotary evaporation. The products were dissolved in CDCl 3 and analysed with [1] HNMR. For the reaction between iodobenzene and PhB(OH) 2 , the percentage yield was calculated by comparing the integration of the peak at δ 7.4 p.p.m. (biphenyl) with that at δ 7.1 p.p.m. (unreacted iodobenzene; Supplementary Fig. 15 ). For coupling of iodotoluene with PhB(OH) 2 , the integration of the peaks at δ 7.5 p.p.m. (4-methylbiphenyl) and δ 6.9 p.p.m. (unreacted iodotoluene) was used to calculate the percent yield ( Supplementary Fig. 10 ). Pd NPs from the aqueous layers were recycled using centrifugation and then dispersed in 1 ml H 2 O. To evaluate the recyclability of catalysts, the reactions were examined by mixing fresh reagents with the recycled Pd NP solutions. Preparation of NovaSyn TGR resin-supported aryl iodide 4-iodobenzoic acid (0.149 g, 0.6 mmol), HOBt·H 2 O (0.092 g, 0.6 mmol) and DIC (94 μl, 0.6 mmol) were pre-mixed in DMF (5 ml) on ice for 1 h. Then, NovaSyn TGR resin 1 (0.48 g, 0.25 mmol g −1 loading) was added ( Supplementary Fig. 11 ). The reaction was conducted by stirring overnight at room temperature. A capping solution consisting of Ac 2 O (45 μl, 0.48 mmol) and pyridine (42 μl, 0.52 mmol) was added, and the reaction was allowed for an additional 30 min. The product, resin 2 ( Supplementary Fig. 11 ), was separated by filtration and washed with DMF (3 × 5 ml), MeOH (3 × 5 ml) and CH 2 Cl 2 (3 × 5 ml) and dried under vacuum. The resin was stored at −20 °C before use. Three-phase test Suzuki coupling reactions were performed under standard condition (0.6 mmol PhB(OH) 2 , 0.3 mmol iodobenzene or iodotoluene, 1 mmol K 2 CO 3 , 10 μg Pd nanocages (0.03 mol%) and 5 ml 80% ethanol aqueous solution) in the presence of resin 2 (42 mg, 0.01 mmol). Reactions were carried out under vigorous stirring at room temperature for iodobenzene and 50 °C for iodotoluene, respectively. After 2 h, the resin was separated by filtration. While the conversion of iodobenzene or iodotoluene in the filtrate was analysed as described in ‘Catalytic Evaluation in Suzuki Coupling Reactions’, the insoluble resins were purified by washing with H 2 O (3 × 2 ml), MeOH (3 × 2 ml), EtOAc (3 × 2 ml), THF (3 × 2 ml) and CH 2 Cl 2 (3 × 5 ml). Here resin 2 would convert to resin 3 if any active homogeneous catalyst appears in the solution during the coupling reaction ( Supplementary Fig. 11 ). This conversion can be verified by analysing the compounds after cleavage with TFA, where 5 and 6 were cleavage products of 2 and 3 , respectively ( Supplementary Fig. 11 ). To this end, the resin was treated with 2 ml 95% v/v TFA in CH 2 Cl 2 for 30 min at room temperature. The cleavage solution was filtrated and the resin was washed with CH 2 Cl 2 (3 × 2 ml), EtOAc (3 × 2 ml) and THF (3 × 2 ml). The combined filtrates were evaporated. The product was dissolved in THF and analysed with GC–MS ( Supplementary Fig. 12 ). In this sample, dodecane was added as an internal standard. The product was also confirmed with [1] HNMR after dissolving in DMSO-d6 ( Supplementary Fig. 13 ). Characterization TEM images were captured on a JEM 2100 microscope (JEOL Inc) with an acceleration voltage of 200 kV. Samples were prepared by drying 2 μl of the NP solution on carbon-coated copper grids under ambient condition. UV–vis absorption spectra were recorded on Beckman Coulter DU 800 UV/Vis Spectrophotometer. 1 HNMR spectra were recorded on Bruke 500 MHz spectrometers. Chemical shifts ( δ values) were reported in p.p.m. downfield from internal tetramethylsilane. How to cite this article: Wei, Z. and Matsui, H. Rational strategy for shaped nanomaterial synthesis in reverse micelle reactors. Nat. Commun. 5:3870 doi: 10.1038/ncomms4870 (2014).